Geographic range did not confer resilience to extinction in terrestrial vertebrates at the end-Triassic crisis Rates of extinction vary greatly through geological time, with losses particularly concentrated in mass extinctions. Species duration at other times varies greatly, but the reasons for this are unclear. Geographical range correlates with lineage duration amongst marine invertebrates, but it is less clear how far this generality extends to other groups in other habitats. It is also unclear whether a wide geographical distribution makes groups more likely to survive mass extinctions. Here we test for extinction selectivity amongst terrestrial vertebrates across the end-Triassic event. We demonstrate that terrestrial vertebrate clades with larger geographical ranges were more resilient to extinction than those with smaller ranges throughout the Triassic and Jurassic. However, this relationship weakened with increasing proximity to the end-Triassic mass extinction, breaking down altogether across the event itself. We demonstrate that these findings are not a function of sampling biases; a perennial issue in studies of this kind. Is it possible to make generalizations about which clades and higher taxa are most likely to go extinct on geological timescales? Geographic range is often claimed to be a determinant of extinction vulnerability [1] , [2] , [3] , [4] , [5] , [6] . Groups with restricted ranges are widely believed to suffer extinction more frequently than those with broader ranges [1] because the latter are thought to be afforded some resilience to regional environmental perturbations [7] , [8] . During global biotic crises, by contrast, there is reasoned to be no such selectivity [2] , [6] since widespread environmental disturbances simultaneously affect both wide- and narrow-ranging taxa on global scales [1] , [3] , [6] . Surprisingly, the effect of geographic range on extinction risk has not been tested comprehensively for the terrestrial fossil record, with a striking paucity of studies on vertebrates of any kind. Most published studies focus on marine invertebrates [3] , [4] , [5] , [6] , [8] , [9] , [10] , and despite geographic range being used as a major criterion for assessing the extinction risk of modern terrestrial species [11] , it is unclear that the findings from these fossil taxa can be extended to all groups in all major habitats. Moreover, little is known about the difference between intervals with background levels of extinction and those characterized as mass extinctions [3] . The only way to answer such questions is to utilize fossil evidence of past organismal distributions [5] , [12] . The Triassic to Jurassic is a critically important period in terrestrial vertebrate evolution [13] , [14] . In particular, it follows the largest of all mass extinctions, the Permo–Triassic ‘great dying’ [13] , [14] , [15] . Many terrestrial vertebrate lineages originated in the aftermath of the Permo–Triassic event, but were subsequently subjected to major changes in terrestrial ecosystems throughout the ensuing Triassic and Jurassic. These changes included the gradual aridification of Pangaea [16] , as well as its initial rifting and fragmentation [17] allied to the eruption of the Central Atlantic magmatic province [18] , [19] . This culminated in the end-Triassic mass extinction event [16] , [20] that saw the demise of numerous amphibian and reptile groups before the subsequent rise to dominance of the dinosaurs [13] , [16] , [21] , [22] , [23] . The significant vertebrate faunal turnover throughout the Triassic and Jurassic (lying either side of the end-Triassic mass extinction) make this an ideal period in which to study extinction selectivity. We therefore collated palaeobiogeographical and stratigraphic distributional data [24] for Triassic and Jurassic terrestrial vertebrate clades to ask three questions. (1) Is there is a relationship between palaeobiogeographical distribution and the risk of extinction during ‘normal’ times? (2) Does any such relationship disappear across the end-Triassic mass extinction? (3) Can any of these findings be attributed to sampling biases? We find that wider geographical range conferred greater resilience to extinction in terrestrial vertebrate groups throughout most of the Triassic and Jurassic. However, this insurance weakened towards the end-Triassic mass extinction, and was imperceptible across the event itself. Major sampling biases were discounted as the cause of these patterns. 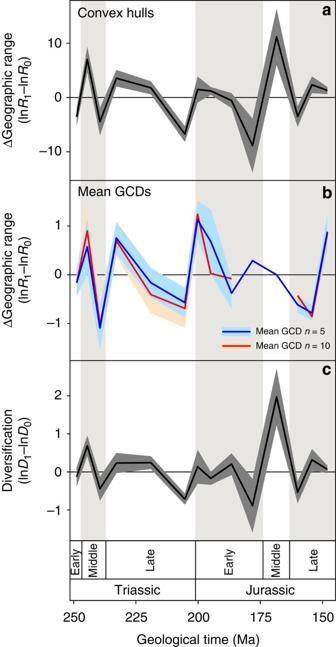Figure 1: Mean rates of change in geographic range size and diversification rates for terrestrial vertebrates, partitioned by time bin. Rate of change in geographic range size (ΔGeographic range) as represented by (a) convex hulls around raw palaeogeographic occurrences and (b) mean GCD between palaeogeographic occurrences standardized to 5 and 10 samples; and (c) mean vertebrate diversification rates of ranged-through diversity data (ΔDiversification). The fossil records of the Ladinian12, Toarcian19and much of the middle Jurassic28,29,30are of lower quality than the rest of Mesozoic, and this may contribute to some of the negative diversity changes therein. The drop in diversity observed through the Rhaetian could also be regarded as a sampling artefact as the Rhaetian is not as well sampled as the preceding Norian. However, the upper Triassic represents one of the highest-quality terrestrial fossil records22,30. Alternating grey and white bars correspond to Triassic–Jurassic epochs. Geographic range and diversification rates are correlated Diversification rates and changes in geographic range at the clade level are positively and strongly correlated across all time bins ( Figs 1 and 2 and Supplementary Table 1 ), with weaker (but still mostly significant) correlations when the data are subdivided into epochs ( Fig. 2 and Supplementary Table 1 ). The strong correlation between changes in geographic range and diversification rate across all time intervals (and at epoch level and within stage-level time bins) confirms that increasing range size coincides with increasing diversity, whilst range size reductions typically attend diversity reductions. Taxa with larger geographic ranges are therefore more likely to exhibit increasing diversity and lower extinction rates than those with smaller ranges. Greater rates of origination might also be expected to result from more extensive ranges; first, because large ranges are more likely to be fragmented into peripheral isolates, and second, because larger ranges encompass a greater diversity of environments and selective forces [25] , [26] . This pattern is the opposite of that proposed for the marine invertebrate fauna, where taxa with narrow ranges show higher origination rates [6] , [27] . The results from our geographic range data sets, both raw convex hull and standardized mean great circle distances (GCDs; Fig. 1 ), are similar, demonstrating that our findings are not contingent on the precise methodology used. Figure 1: Mean rates of change in geographic range size and diversification rates for terrestrial vertebrates, partitioned by time bin. Rate of change in geographic range size (ΔGeographic range) as represented by ( a ) convex hulls around raw palaeogeographic occurrences and ( b ) mean GCD between palaeogeographic occurrences standardized to 5 and 10 samples; and ( c ) mean vertebrate diversification rates of ranged-through diversity data (ΔDiversification). The fossil records of the Ladinian [12] , Toarcian [19] and much of the middle Jurassic [28] , [29] , [30] are of lower quality than the rest of Mesozoic, and this may contribute to some of the negative diversity changes therein. The drop in diversity observed through the Rhaetian could also be regarded as a sampling artefact as the Rhaetian is not as well sampled as the preceding Norian. However, the upper Triassic represents one of the highest-quality terrestrial fossil records [22] , [30] . Alternating grey and white bars correspond to Triassic–Jurassic epochs. 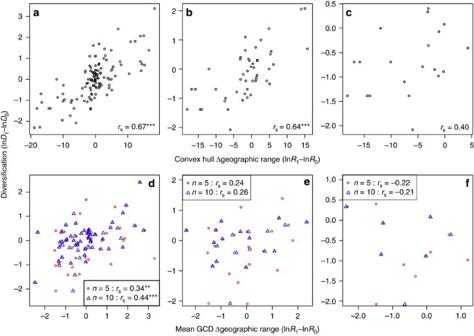Figure 2: Scatter plots of diversification rates against per lineage rates of change in geographic range size. Rate of geographic range size change (ΔGeographic range) as calculated using convex hulls around raw occurrence data for (a) all time bins, (b) late Triassic and (c) Rhaetian. Rate of geographic range size change calculated as mean GCDs between occurrences standardized to samples of 5 and 10 occurrences for (d) all time bins, (e) late Triassic and (f) Rhaetian. Spearman’s rank correlation coefficients **significant atP<0.01, ***significant atP<0.001. Full size image Figure 2: Scatter plots of diversification rates against per lineage rates of change in geographic range size. Rate of geographic range size change (ΔGeographic range) as calculated using convex hulls around raw occurrence data for ( a ) all time bins, ( b ) late Triassic and ( c ) Rhaetian. Rate of geographic range size change calculated as mean GCDs between occurrences standardized to samples of 5 and 10 occurrences for ( d ) all time bins, ( e ) late Triassic and ( f ) Rhaetian. Spearman’s rank correlation coefficients **significant at P <0.01, ***significant at P <0.001. Full size image This relationship breaks down across the mass extinction Strikingly, rates of geographic range change and diversification are not significantly correlated immediately before the end-Triassic extinction (during the Rhaetian), whereas this correlation is significant even in the Carnian and Norian stages that immediately precede it ( Fig. 2 and Supplementary Table 1 ). Hence, diversification rate becomes decoupled from range size change rate across the extinction boundary and the insurance against extinction offered by larger geographic ranges at other times disappears. During the end-Triassic mass extinction event, relatively widespread groups are as likely to suffer high levels of extinction as groups with narrower geographic ranges. For example, Phytosauria and Theropoda have similar, geographic ranges in the Rhaetian ( Fig. 3 ). However, phytosaurs suffer complete extinction at the end Triassic, whereas theropod diversity remains stable across the boundary and into the Hettangian, even whilst undergoing significant range expansion ( Fig. 3 ). Of the time intervals that do not show significant correlation between diversification rate and geographic range change rate, all have very small sample sizes apart from the Rhaetian. The standardized mean GCD range metrics show less correlation with diversification rate than the raw convex hull metric ( Supplementary Table 1 ). This is unsurprising since a reduced sample size leads to a reduction in statistical power. However, many of these nonsignificant correlations still have relatively high correlation coefficients and are approaching significance, whereas the Rhaetian results are clearly different (with negative coefficients that are far from significant) ( Supplementary Table 1 ). Our temporal divisions are very much longer (2.0–18.9 Myrs) [28] , [29] than the extinction event [20] , which occurred in pulses over a period of <1.0 Myr (ref. 19 ). Effects are therefore time averaged, meaning that the breakdown of the relationship between diversification rate and the rate of geographic range change in the very end Triassic (an interval known to contain a major biotic crisis) is even more striking. 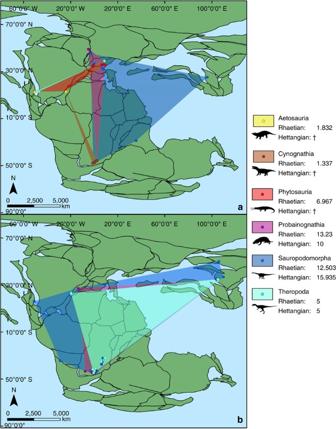Figure 3: Geographic range maps before and after the end-Triassic mass extinction. Convex hull geographic range maps and mean generic diversity of six terrestrial vertebrate groups during the (a) Rhaetian and (b) Hettangian. The Aetosauria, Cynognathia and Phytosauria became extinct during the biotic crisis, despite the widespread distribution of Cynognathia and Phytosauria in the Rhaetian. The Probainognathia, Sauropodomorpha and Theropoda all survived the biotic crisis and expanded their ranges in the Hettangian, albeit with different diversification trajectories. The diversity of Sauropodomorpha increased, the diversity of Theropoda was stationary and that of Probainognathia decreased across the boundary. Figure 3: Geographic range maps before and after the end-Triassic mass extinction. Convex hull geographic range maps and mean generic diversity of six terrestrial vertebrate groups during the ( a ) Rhaetian and ( b ) Hettangian. The Aetosauria, Cynognathia and Phytosauria became extinct during the biotic crisis, despite the widespread distribution of Cynognathia and Phytosauria in the Rhaetian. The Probainognathia, Sauropodomorpha and Theropoda all survived the biotic crisis and expanded their ranges in the Hettangian, albeit with different diversification trajectories. The diversity of Sauropodomorpha increased, the diversity of Theropoda was stationary and that of Probainognathia decreased across the boundary. Full size image Sampling biases have little effect on our results We observed several significant bivariate correlations between diversification rate, geographic range change rate and various putative sampling proxies detrended using first differences ( Supplementary Tables 2 and 3 ). However, multiple regression models identified the changes in geographic range rate as the dominant variable influencing diversification rate ( Table 1 and Supplementary Tables 4–9 ). Table 1 Summary of multiple regression models of diversity change (dependent variable) in terms of geographic range change and sampling and environmental proxies. Full size table Although certain parts of the Triassic–Jurassic are reputed to have a poor terrestrial fossil record (that is, Ladinian, Toarcian–mid Jurassic) [13] , [20] , [30] , [31] , [32] , the late Triassic possesses one of the best [23] , [32] ( Fig. 4 ). We see positive correlations between land area and geographic range and a negative correlation between sea level and range in the GCD data, but also positive correlations between sea level and geographic range and between sea level and diversification rate in the convex hull data. This suggests that greater land area and lower sea levels may result in greater geographic ranges amongst terrestrial organisms. However, the negative correlation between standardized range and sea level (and the lack of correlation between diversification rate and land area) suggests that while expanding landmasses might be expected to induce the expansion of terrestrial ranges and increase diversification, climatic and other effects complicate this relationship. Indeed, the typically harsh environments in deep continental interiors may constrain many ranges. Specifically, lethally hot temperatures, particularly in the early Triassic, may have limited or even excluded diversity in equatorial regions [33] . Individual lineage ranges correlate with total ranges across time bins, and both appear to reflect the same underlying pattern. The considerable variation between individual lineage ranges within each bin (coupled with the fact that the standardized range metrics still show some correlation with total range, albeit weaker than the raw range metrics) indicates that range estimates are not governed straightforwardly by sampling intensity ( Figs 1 and 3 ). Moreover, the absence of terrestrial vertebrates from equatorial regions is entirely plausible during the climatic greenhouse of the early Triassic [33] . Groups with broader geographical distributions are likely to be subject to a wider range of selective pressures and the peripheral isolation of subgroups; both factors favouring speciation and increasing diversity [25] , [26] . However, the weak correlation observed between changes in fossil abundance and both diversification rate and geographic range change may be representative of sampling bias. It is also possible that a greater investment of research effort in more abundant fossil groups may have resulted in increased taxonomic splitting [34] . 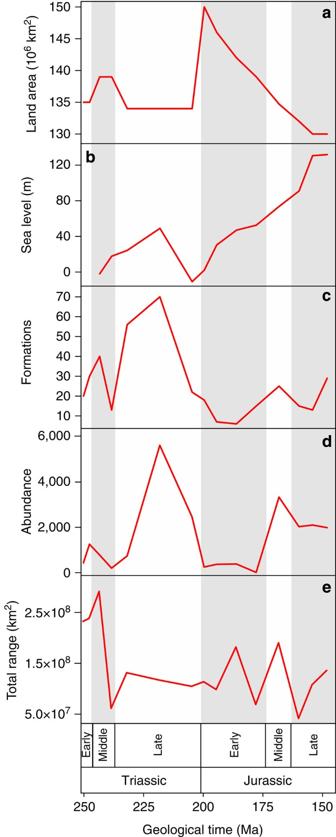Figure 4: Sampling and environmental proxy data. (a) Non-marine area58, (b) average sea level60, (c) terrestrial formation count24, (d) fossil abundance24and (e) total geographic range of all taxa. Alternating grey and white bars correspond to Triassic–Jurassic epochs. Figure 4: Sampling and environmental proxy data. ( a ) Non-marine area [58] , ( b ) average sea level [60] , ( c ) terrestrial formation count [24] , ( d ) fossil abundance [24] and ( e ) total geographic range of all taxa. Alternating grey and white bars correspond to Triassic–Jurassic epochs. Full size image We also observed significant pairwise correlations between both raw and standardized geographic range change and diversification rate on one hand, and changes in numbers of formations on the other. Although formation counts are regarded as effective sampling proxies for terrestrial data sets [35] , redundancy between sampling proxies and diversity metrics (arising from the probable non-independence of formation and fossil content) remains problematic [36] , [37] , [38] . In practice, the level of this redundancy is likely to be minimized by the use of all terrestrial vertebrate-bearing formations [39] , [40] , rather than by adopting a stricter count of only those formations containing a particular group of terrestrial vertebrate fossils [31] , [41] , [42] , [43] . However, standardization of geographic range data results in the removal of significant correlations between range size and fossil abundance, coupled with a weakening of the correlation between range size and total range size (that is, standardizing geographic range calculations to a constant sample size across all lineages in each time bin appears to remove putative sampling effects). By contrast, standardizing range data does not affect the correlation between range size and formation counts. This last relationship may therefore arise from redundancy [36] , rather than being a temporal bias resulting from variation in the amount of preserved sedimentary rock (and concomitant intensity of sampling) through geological time. The multiple regression models show that geographic range change is the dominant driver of diversification rate through the Triassic–Jurassic, to the exclusion of all the sampling proxies in the model using convex hulls, but with total range and sea level showing some influence in the standardized mean GCD models. This suggests that, although sampling biases are a perennial issue in fossil data sets, the link between changes in geographic range and diversification rate appear robust, despite the patchy nature of the vertebrate fossil record. Implications for extinction studies We demonstrate that broad geographic range conferred insurance against extinction on major clades of terrestrial vertebrates during periods with background levels of extinction. In line with marine invertebrate studies across the same biotic crisis [6] and at other times in the Phanerozoic [3] , this insurance disappeared during the end-Triassic mass extinction. However, these results are in marked contrast to patterns reported for marine invertebrates at the Cretaceous–Paleogene extinction [9] , [44] (where groups with larger geographic ranges retain increased resilience to extinction across the crisis than those with smaller ranges). It is reasonably common to observe discrete macroevolutionary patterns in different higher taxa or across different major habitats. Notable examples include the incongruence between terrestrial and marine Phanerozoic diversity curves [45] , [46] , [47] , variations in the apparent force of Cope’s rule sensu lato in different higher taxa [48] , [49] , [50] , and variations in the relationships between body size, population density and fecundity across clades [51] , [52] . However, the differences between patterns observed at major extinction events may result from differences between the particular driving forces of the crises themselves. These differences highlight the need for greater numbers of large-scale, comparative studies before attempting to make macroevolutionary generalizations. Fortunately, the expansion and refinement of resources such as the Paleobiology Database, coupled with quantitative tools such as GIS, have great potential for testing temporal and spatial macroevolutionary patterns. Equally, palaeontological data provide a broader perspective on the current biodiversity crisis. Specifically, it enables deep time tests of the purported relationships between present day extinction susceptibility and geographical range size [53] , [54] , latitudinal distribution [55] , niche breadth [56] and body size [57] , [58] . Fossil occurrence data Stage-level occurrence data for Triassic–Jurassic terrestrial vertebrates were initially downloaded from the Paleobiology Databse [24] ( https://paleobiodb.org ) on 4 February 2013 (last accessed 20 April 2015) and, after preprocessing, consisted of 3,507 occurrences of 857 genera (see Supplementary Note 1 for Paleobiology Database download specifications). Terrestrial vertebrate occurrences from marine deposits were not included as they would not give a true representation of geographic range. Ichnogenera and other form taxa where then removed from the data set as they could not be assigned accurately to parent genera. Marine tetrapod taxa recorded in terrestrial formations were also removed. Generic indeterminate taxa and taxa with uncertain generic assignments (that is, aff. , cf. , ex gr. , sensu lato , ?) were also excluded. Although these exclusions inevitably resulted in an underestimation of the geographic range of higher taxonomic groups, it would be inappropriate to compare ranges constructed from taxa of uncertain affiliation with rates of generic extinction, origination and diversification, which cannot include these indeterminate occurrences. Fossil occurrences were vetted for synonymy and outdated taxonomy, and sorted into higher taxonomic groups according to phylogenetic and ecological relationships within the constraints of reasonable sample sizes (see Supplementary Note 1 for detailed classification of taxa). As with all higher taxonomic classification, groups were not directly comparable. This is an unavoidable problem unless working at the species or, to a lesser extent, the generic level. Two data sets were compiled: data 1 and data 2 ( Supplementary Fig. 1 ). Data 1 ( Supplementary Data 1 ) contained a number of paraphyletic assemblages where basal taxa of particular lineages were grouped together to form a paraphyletic ‘stem’ assemblage (for example, Archosauriformes, basal Cynodontia and Dinosauromorpha; Supplementary Fig. 1 ). Since the inclusion of paraphyletic groups is arguably problematic (they do not represent ‘true’ evolutionary groups), a second data set excluding all parapyla was also prepared. In data 2 , the paraphyletic assemblages were collapsed into smaller, monophyletic family-level groups wherever possible ( Supplementary Fig. 1 ). The two data sets correlated very closely in terms of both geographic range change rate and diversification rate. All analyses in the manuscript therefore refer exclusively to data 1 . Fossil occurrences were binned at the stratigraphic stage level. Any occurrences not assigned to a stage were attached to the stage, or range of stages, corresponding to the formation from which they were recovered. Fossil occurrences that were assigned to more than one stage were randomly assigned to a single stage within their given range, a process that was repeated 1,000 times to obtain a mean value. This method avoided either the artificial inflation or deflation of taxonomic richness in any given stage compared with maximum or minimum diversity values. Sampling and environmental proxy data Non-marine area . A mean estimate of the continental landmass for each stage [59] . It was anticipated that geographic range would correlate positively with land area as the area of terrestrial habitat creates an upper limit for the geographic range of terrestrial organisms. These measurements were derived from an independent source [59] , and were subject to different definitions of stage-level boundaries than the fossil occurrence data set, which used the Geological Time Scale 2012 (ref. 60 ). Sea level . A mean estimate of relative sea level for each stage [61] . It was expected that geographic range would correlate inversely with mean sea level, as higher sea level would result in less terrestrial landmass for terrestrial organisms to inhabit. As with the non-marine area measurements, the sea level averages were obtained from an independent source [61] and are subject to different definitions of stage-level boundaries from the fossil occurrence data set [60] . Terrestrial formations . Formation counts are widely regarded as effective sampling proxies for the terrestrial fossil record [24] , [31] , [35] , [42] , [62] . It is still unclear if this is true, as formation counts probably share a common signal with fossil occurrence data (that is, formations are not independent from their fossil content [36] , [37] ). However, given the lack of comprehensive data on global sedimentary rock outcrop area, formation counts offer the only possible metric of global rock availability. In this analysis, redundancy was minimized by using a total count of terrestrial tetrapod bearing formations, rather than a strict count of group-specific bearing formations. There is also an argument for redundancy between formation counts and geographic range, as a taxon that is genuinely wide ranging is more likely to be present in more formations across the globe than a taxon with a small geographic range. Such possibilities were explored using multiple regression models. Fossil abundance . The fossil abundance per time period serves as a proxy for human sampling and collecting effort [24] . However, there is danger of circularity, as palaeontologists will be more likely to collect from formations yielding a higher number of fossils [38] , [63] . Therefore, fossil abundance may be more representative of preservational factors or true biological abundance, rather than a measure of human sampling effort. Total geographic range . It is reasonable to assume that vertebrates were not genuinely absent from large areas of the globe through parts of the Triassic–Jurassic. Therefore, if total geographic range (that is the total geographic range of all tetrapod occurrences per time bin) were to correlate strongly with the geographic ranges of individual fossil groups, it would indicate that the pattern of geographic range through the study period is controlled by spatial sampling rather than reflecting a biological pattern. Analysis Palaeogeographic ranges were constructed by converting modern fossil occurrence coordinates to palaeocoordinates using PointTracker [64] . Palaeogeographic ranges were constructed using two methods: (i) in ArcGIS v10.1 using convex hulls around the palaeogeographic occurrences for each group [65] , [66] ; and (ii) using mean GCDs between palaeogeographic occurrences with sample sizes standardized to 5 and 10 occurrences per lineage per time bin and replicated 1,000 times to obtain a mean value. GCD distances were calculated using the spherical law of cosines (as an acceptable approximation of the Haversine formula for terrestrial calculations). Per lineage origination ( O r ) and extinction ( E r ) rates were calculated using the methodology of Foote [67] and modified by Foote [68] : where N bt =number of range-through taxa, N ft =number of taxa that originate within time bin and cross top boundary of time bin and N bL =number of taxa that cross bottom boundary of time bin but make their last appearance in time bin. Rates were not expressed relative to time bin duration; although this may cause underestimation of rates in shorter time bins relative to longer time bins, Foote [28] demonstrated that both extinction and origination are pulsed rather than spread throughout time intervals. All analyses were carried out at the generic level. No significant correlations were detected between geographic range change and extinction rate or between geographic range change and origination rate ( Supplementary Table 10 ). The absence of significant correlations between origination/extinction rates and change in geographic range could be regarded as somewhat surprising, but this result is a function of the paucity of data for the rate calculations. However, the extinction and origination rate calculations rely on taxa that range through three consecutive time bins [67] , which are scarce in this data set because of the patchiness of the terrestrial fossil record and the long durations of the time bins. Therefore, it was judged that a metric of diversification calculated from generic range data offered a more robust picture of biotic change. Diversification rate ( D r ) and geographic change rate ( R r ) were calculated using a metric modified from Rode and Lieberman [69] : where D 1 =ranged-through diversity calculated from first and last appearances for current time interval, D 0 =ranged-through diversity calculated from first and last appearances for the previous time interval, R 1 =geographic range in time interval and R 0 =geographic range in previous time interval. Relationships between geographic range change and generic diversification rates within clades were tested using pairwise Spearman’s rank–order correlation tests. Putative sampling biases were investigated using both pairwise correlation and multiple regression models, with diversification rate as the dependent variable and geographic range and various sampling proxies as independent variables. First differencing was used to detrend the sampling proxy data before comparison with the biotic rate data. All statistical analyses were carried out in R 3.1.1. How to cite this article: Dunhill, A. M. et al. Geographic range did not confer resilience to extinction in terrestrial vertebrates at the end-Triassic crisis. Nat. Commun. 6:7980 doi: 10.1038/ncomms8980 (2015).